FBH1 influences DNA replication fork stability and homologous recombination through ubiquitylation of RAD51 Unscheduled homologous recombination (HR) can lead to genomic instability, which greatly increases the threat of neoplastic transformation in humans. The F-box DNA helicase 1 (FBH1) is a 3′–5′ DNA helicase with a putative function as a negative regulator of HR. It is the only known DNA helicase to contain an F-box, suggesting that one of its functions is to act as a ubiquitin ligase as part of an SCF (SKP1, CUL1 and F-box) complex. Here we report that the central player in HR, RAD51, is ubiquitylated by the SCF FBH1 complex. Expression of an ubiquitylation-resistant form of RAD51 in human cells leads to hyperrecombination, as well as several phenotypes indicative of an altered response to DNA replication stress. These effects are likely to be mediated by the enhanced nuclear matrix association of the ubiquitylation-resistant RAD51. These data are consistent with FBH1 acting as a negative regulator of RAD51 function in human cells. Faithful DNA replication is essential for cell proliferation. Nevertheless, a number of circumstances can arise in cells that lead to the stalling or collapse of DNA replication forks. On short-term replication blockage, such as following exposure of cells to the ribonucleotide reductase inhibitor, hydroxyurea (HU), the replication machinery is stalled, but remains bound to the DNA [1] . If the duration of replication stalling is prolonged, the replisome components can detach from the stalled fork, and the exposed fork can be processed into a double-strand break (DSB). This fork breakage process is most probably mediated by the DNA structure-specific endonuclease MUS81-EME1 (ref. 2 ). Under these circumstances, the fork is deemed to have ‘collapsed’. Stalled and collapsed forks both require the protective function of the RAD51 recombinase, but different roles of RAD51 are apparently required in each case. In the case of a stalled fork, RAD51 serves to stabilize the fork, in a process that does not appear to require the canonical homologous recombination (HR) machinery. In this pathway, RAD51 has been proposed to coat the single-stranded DNA (ssDNA) region adjacent to the stalled fork, potentially facilitating the formation of a Holliday junction via so-called fork regression (reversal), which involves the annealing of the two nascent DNA strands [3] . Indeed, the RAD51 homologue in Escherichia coli , RecA, has been demonstrated to promote this process in vitro [4] . In addition, RAD51 has been reported to protect the nascent DNA from MRE11-mediated degradation at stalled replication forks [5] , [6] . In contrast to this HR-independent function of RAD51, the canonical HR pathway is known to operate at collapsed forks, where a DSB is generated. One of the key steps in repair of the single-ended DSB formed at a collapsed fork is the formation of a RAD51 protein filament on the ssDNA generated by DSB end resection. This nucleoprotein filament is required for the search for a homologous DNA sequence and for repair of the break [7] . RAD51 is also involved in the reassembly of key DNA replication proteins, including the so-called CMG complex comprising CDC45-MCM-GINS, after replication forks have collapsed [8] . Despite this protective role of RAD51 and HR factors more generally at stalled/collapsed replication forks, it is clear that uncontrolled HR can lead to genome rearrangements and loss of heterozygosity, which are potent drivers of tumorigenesis [9] . As RAD51 is a key player in replication-associated HR, controlling the binding of RAD51 to its potential DNA substrates or to chromatin more generally would be an effective means to regulate the balance between the beneficial and detrimental roles of HR in an effort to preserve genome stability. Several DNA helicases have been identified that can control the stability of a RAD51 nucleoprotein filament [10] , [11] , [12] , [13] . Many of these belong to the UvrD family of proteins, such as Srs2 in yeast and PARI in mammals [12] , [13] , [14] . Mammalian cells express another UvrD family member, FBH1 (F-box DNA helicase 1), which has been reported previously to suppress HR [15] . FBH1 is conserved in human, mouse and Schizosaccharomyces pombe cells, but is not found in Saccharomyces cerevisiae [16] . In addition to the helicase domain, there is an amino-terminal F-box domain present in FBH1. F-box proteins form part of the so-called SCF complexes (SKP1-CUL1-F-box protein), which generally act as E3 ubiquitin ligases [17] . Ubiquitylation is a posttranslational modification that leads to the covalent attachment of the ubiquitin peptide to particular lysine residues in the target protein. This modification may regulate the substrate’s function or target the substrate for proteasomal degradation [17] . Previous data derived from studies in S. pombe have suggested that both the F-box domain and the helicase domain of Fbh1 are required for the repair of DNA damage in that organism, although the helicase function seems more critical [18] , [19] . Moreover, genetic analysis suggested that yeast Fbh1 acts downstream of Rad51 in the HR pathway [18] , [20] . Consistent with this, the level of Rad51 nuclear foci is greatly increased in Fbh1-deficient yeast, a phenotype that is also characteristic of FBH1-depleted human cells [15] , [21] , [22] . Recently, we found that the helicase function of FBH1 co-operates with the MUS81-EME1 nuclease in generating DSBs following replication stress induced by HU [23] . FBH1 is often mutated in melanoma cells, which suggests that the DSBs generated in this context by the action of FBH1 might serve to trigger apoptosis, to prevent oncogenic transformation [24] , [25] . Interestingly, human and mouse cells expressing a helicase-dead version of FBH1 are resistant to the cytotoxic effects of replication stress induced by HU [23] . In addition, FBH1 forms HU-induced nuclear foci that co-localize with the ssDNA-binding protein, RPA [15] . These observations strongly implicate the helicase function of FBH1 in coping with some aspect of DNA replication stress. Consistent with this, recent data indicate that human FBH1 can displace RAD51 filaments from ssDNA [22] . However, the role of the F-box domain of FBH1 remains undefined. Although UvrD family helicases are implicated in the regulation of RAD51 function in a diverse range of cell types, it is not clear whether the F-box also plays a role in regulating RAD51 or HR more generally in mammalian cells. Indeed, it has been reported that an F-box-mutated variant of S. pombe Fbh1 is largely functional, which implies the F-box may only play a minor role in HR and in the cellular response to replication problems in that organism [18] . In human cells, the substrate of the FBH1 ubiquitylation and the role of the F-box in pathways for coping with replication stress are currently unknown. Here we have addressed these issues. We demonstrate that RAD51 can be ubiquitylated by the SCF FBH1 complex in vitro . In cells expressing an ubiquitylation-resistant form of RAD51, the RAD51 protein shows enhanced chromatin association during replication stress. In these cells, the frequency of replication fork stalling is reduced, while recovery of replication following replication stress is enhanced. These cells also show increased resistance to replication inhibitors, and hyperrecombination, consistent with a role for FBH1 in regulating RAD51 function in human cells. RAD51 is ubiquitylated by the SCF FBH1 complex in vitro The FBH1 protein is implicated in the control of RAD51 function, most probably in the context of stalled or damaged DNA replication forks. Although the helicase function of FBH1 is thought to regulate the stable association of RAD51 with DNA, the role of the F-box domain in FBH1 has not been defined. To investigate the function of the F-box, we purified recombinant human FBH1, together with the other SCF complex components, as well as human RAD51 protein ( Supplementary Fig. 1a,b ). The purified SCF FBH1 complex was then tested for its ability to ubiquitylate the purified RAD51 protein in vitro . In the presence of SCF FBH1 and ubiquitin, a new species of the RAD51 protein (which normally migrates at 37 kDa on SDS–polyacrylamide gel electrophoresis (PAGE)) was observed with a migration equivalent to 50 kDa ( Fig. 1a ). This would be consistent with the addition of a single ubiquitin moiety to the RAD51 protein. To confirm that this protein modification was via ubiquitylation, we repeated the reactions using haemagglutinin (HA) epitope-tagged ubiquitin instead of untagged ubiquitin. In this case, the modified RAD51 showed a further reduction in mobility on SDS–PAGE due to the presence of the HA tag ( Fig. 1a ). Hence, we conclude that SCF FBH1 can ubiquitylate RAD51 in vitro . This modification required, as expected, an E1 enzyme and an E2 enzyme ( Supplementary Fig. 1c ), but occurred independently of the presence or absence of ssDNA ( Fig. 1b ). A negative control reaction is shown in Fig. 1d described below, to demonstrate a requirement for ubiquitin itself. The preferred E2 appeared to be UbcH5a, which could not be replaced by Cdc34 or UbcH6 ( Supplementary Fig. 1c,d ). The reaction was also not stimulated by the presence of Nedd8 ( Supplementary Fig. 1c ). To assess whether there was any specificity to the reaction, we replaced RAD51 with RPA, FANCD2 or BLM protein. In none of these cases could we detect ubiquitylation by the SCF FBH1 complex ( Supplementary Fig. 1e ). 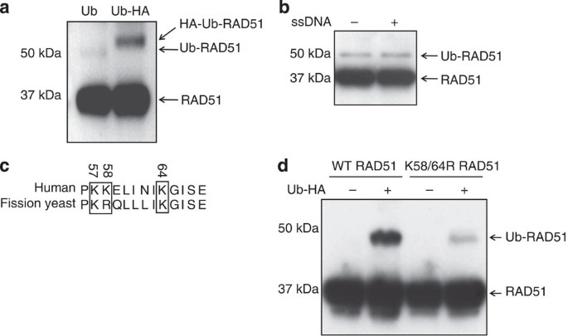Figure 1: RAD51 is ubiquitylatedin vitroby FBH1. (a) Western blotting of products from ubiquitylation of RAD51 by SCFFBH1probed with an anti-RAD51 antibody. The positions of the unmodified RAD51, the ubiquitylated RAD51 (ub-RAD51) and the HA-Ub RAD51 are shown on the right. (b) The ubiquitylation of RAD51 by SCFFBH1has no requirement for ssDNA. (c) Protein sequence alignment of a region of the human andS. pombeRAD51 proteins. The conserved lysines/arginines are bracketed and their positions are numbered above. (d) WT RAD51 or RAD51 containing mutations of lysines to arginines on position 58 and 64 (K58/64R) were subjected toin vitroubiquitylation by SCFFBH1. The+and −symbols denote the presence or absence of the indicated protein, respectively. A western blot is shown of the products of the assay probed with an anti-RAD51 antibody. Figure 1: RAD51 is ubiquitylated in vitro by FBH1. ( a ) Western blotting of products from ubiquitylation of RAD51 by SCF FBH1 probed with an anti-RAD51 antibody. The positions of the unmodified RAD51, the ubiquitylated RAD51 (ub-RAD51) and the HA-Ub RAD51 are shown on the right. ( b ) The ubiquitylation of RAD51 by SCF FBH1 has no requirement for ssDNA. ( c ) Protein sequence alignment of a region of the human and S. pombe RAD51 proteins. The conserved lysines/arginines are bracketed and their positions are numbered above. ( d ) WT RAD51 or RAD51 containing mutations of lysines to arginines on position 58 and 64 (K58/64R) were subjected to in vitro ubiquitylation by SCF FBH1 . The+and −symbols denote the presence or absence of the indicated protein, respectively. A western blot is shown of the products of the assay probed with an anti-RAD51 antibody. Full size image Identification of the sites of ubiquitylation on RAD51 A previous proteome-wide mass spectrometry study identified K58 and K64 on RAD51 as being ubiquitylated in human cells [26] . To identify whether these lysine residues could be targeted by SCF FBH1 , we subjected the in vitro ubiquitylated RAD51 to mass spectrometry following trypsin digestion. This analysis provided 79% sequence coverage of RAD51. Five modified residues were identified within the population of RAD51 protein molecules, of which the most prominent were K58 and K64 ( Supplementary Table 1 ). K58 and K64 are in the N-terminal domain of RAD51, which lies outside of the core ‘RecA-like’ ATPase domain. Nevertheless, the region of RAD51 around K58/64 is conserved ( Fig. 1c ), despite the lack of overall conservation of the N-terminal domains of eukaryotic RAD51 proteins. To investigate the importance of the K58/64 residues in the modification of RAD51 by SCF FBH1 , we purified a version of RAD51 containing arginine substitutions of K58 and K64. This protein, designated K58/64R RAD51, possessed a similar ability to interact physically with GST-FBH1 as did the WT RAD51 ( Supplementary Fig. 1f ). However, K58/64R RAD51 was ubiquitylated much less efficiently by FBH1 in vitro than was wild-type (WT) RAD51 ( Fig. 1d ), confirming that the primary sites of modification by FBH1 on RAD51 are K58 and K64. Role of RAD51 ubiquitylation in human cells Next, we investigate the role of K58/64 modification of RAD51 in human cells. To do this, we compared the phenotype of U2OS cells expressing either WT RAD51 or K58/64R RAD51. We reasoned that a ubiquitylation-resistant form of RAD51 might potentially escape the control imposed by FBH1, and therefore be dominantly acting even in cells expressing endogenous RAD51. We focused on the cellular response to replication stress, because our previous studies indicated that FBH1-deficient mouse embryonic stem (ES) cells are abnormally resistant to HU-induced replication fork perturbation [23] . This resistance is manifested both as an increase in clonogenic survival after HU treatment and a decrease in DSB induction compared with WT cells. To analyse the effects of K58/64 ubiquitylation, we generated stable transfectants of U2OS cells expressing either WT or K58/64R RAD51. The level of transfected RAD51 was equal in both cases, and was in excess over that of the endogenous RAD51 by approximately twofold ( Fig. 2a ). Despite lacking any additional tag (because tags are known to adversely affect RAD51 function), the transfected RAD51 had a slightly slower mobility on SDS–PAGE compared with the endogenous protein. This phenomenon has been observed in a previous study [27] . Confirmation that the protein species recognized by this antibody were all RAD51 came from analysis and cells exposed to a small interfering RNA (siRNA) targeted to the coding region of RAD51. After transfection of this siRNA, the level of the endogenous and transfected RAD51 was diminished greatly ( Fig. 2a ). 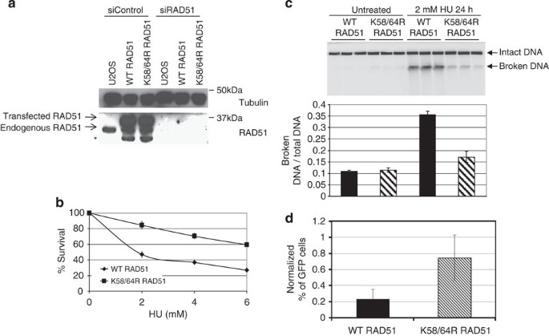Figure 2: Expression of K58/64R RAD51 influences the cellular response to HU. (a) Western blotting of cells transfected with empty vector or a construct expressing either WT RAD51 or K58/64R RAD51, as indicated above the lanes. The set of three samples on the right were derived from cells treated with an siRNA targeted against the coding region ofRAD51, to demonstrate the specificity of the antibody. The positions of the transfected and endogenous RAD51 species are indicated on the left. Tubulin was used as a loading control. The asterisk marks degradation products of RAD51, which were reported previously48. (b) Clonogenic survival curves following exposure of WT RAD51- and K58/64R RAD51-expressing cells to HU, as indicated in the key. Points represent the mean of three independent determinations. (c) Induction of DSBs by treating cells with 2 mM HU for 24 h. The upper panel shows a representative pulsed field gel with triplicate samples for each, while the lower panel shows data for the average of three independent experiments. Bands were quantified by using ImageJ software. (d) Hyperrecombination in K58/64R RAD51-expressing cells as determined by using the DR-GFP assay. The percentage of cells expressing GFP was normalized to a control (a plasmid expressing RFP under the control of the same promoter). The means for two independent experiments are shown. Error bars represent s.d. Figure 2: Expression of K58/64R RAD51 influences the cellular response to HU. ( a ) Western blotting of cells transfected with empty vector or a construct expressing either WT RAD51 or K58/64R RAD51, as indicated above the lanes. The set of three samples on the right were derived from cells treated with an siRNA targeted against the coding region of RAD51 , to demonstrate the specificity of the antibody. The positions of the transfected and endogenous RAD51 species are indicated on the left. Tubulin was used as a loading control. The asterisk marks degradation products of RAD51, which were reported previously [48] . ( b ) Clonogenic survival curves following exposure of WT RAD51- and K58/64R RAD51-expressing cells to HU, as indicated in the key. Points represent the mean of three independent determinations. ( c ) Induction of DSBs by treating cells with 2 mM HU for 24 h. The upper panel shows a representative pulsed field gel with triplicate samples for each, while the lower panel shows data for the average of three independent experiments. Bands were quantified by using ImageJ software. ( d ) Hyperrecombination in K58/64R RAD51-expressing cells as determined by using the DR-GFP assay. The percentage of cells expressing GFP was normalized to a control (a plasmid expressing RFP under the control of the same promoter). The means for two independent experiments are shown. Error bars represent s.d. Full size image Next, we investigated the phenotypic affects of the transfected K58/64R RAD51. Consistent with previous data indicating that FBH1 gene mutation confers resistance to HU, we found that the cells expressing K58/64R RAD51 were significantly more HU resistant than the isogenic control cells expressing WT-transfected RAD51 ( Fig. 2b ; P <0.05 using an unpaired t -test). In cells expressing K58/64R RAD51, the HU resistance was also significant when the endogenous RAD51 protein was depleted using an siRNA targeting the 3′-untranslated region (3′-UTR) of RAD51 , a region of the RAD51 gene that is absent from the transfected RAD51 complementary DNAs ( Supplementary Fig. 2a,b ). These data argue that the endogenous RAD51 does not interfere with the ‘dominant’ phenotypic effects seen when expressing ubiquitylation-resistant RAD51. Moreover, pulsed-field gel electrophoresis analysis indicated that the K58/64R RAD51-expressing cells accumulated significantly fewer DNA DSBs than did the WT RAD51-expressing cells following a 24-h exposure to HU ( Fig. 2c ; P <0.05 using an unpaired t -test). In cells expressing K58/64R RAD51, there was also a diminution in the level of DNA DSBs following HU treatment when the endogenous RAD51 was depleted by an siRNA targeting the 3′-UTR of RAD51 ( Supplementary Fig. 2c ). This difference in DSB levels required that the cells be subjected to prolonged HU treatment, and was much less evident after only a 12-h exposure to HU ( Supplementary Fig. 2d ). Interestingly, we found that the resistance to replication stress in K58/64R RAD51-expressing cells was not limited to HU, but was also seen with aphidicolin, which acts via a different mechanism from HU (direct polymerase inhibition, not dNTP depletion) ( Supplementary Fig. 2e ). However, the K58/64R RAD51-expressing cells were not hyperresistant to ionizing radiation ( Supplementary Fig. 2f ), suggesting a role for RAD51 ubiquitylation only during the cellular response to DNA replication stress. Loss of FBH1 helicase function in mouse ES cells leads to spontaneous hyperrecombination, presumably because RAD51 escapes the normal control imposed by FBH1 (ref. 22 ). Using the widely used and previously validated direct repeat-green fluorescent protein (DR-GFP) assay [28] , we found that the U2OS cells expressing K58/64R RAD51 also showed an approximately threefold increase in the level of recombination compared with control cells expressing WT RAD51 only ( Fig. 2d ; P <0.05 using an unpaired t -test). In cells expressing K58/64R RAD51, the level of recombination was also significantly higher when the endogenous RAD51 was depleted by an siRNA targeting the 3′-UTR of RAD51 (approximately fourfold; Supplementary Fig. 2g,h ). Next, we investigated whether cells expressing either WT or K58/64R RAD51 responded differently following release from prolonged HU-induced arrest. To do this, the DNA fibre technique was employed to quantify replication dynamics. Active replicons were initially labelled by incorporation of CldU and then replication was arrested by exposure of cells to HU. Following removal of the HU, the ability of the cells to recover productive DNA replication was monitored by incorporation of IdU. Three categories of replication were quantified, as depicted in Fig. 3a : (i) irreversibly stalled forks (CldU tracts only; marked in red); (ii) forks that were competent to restart after HU exposure (adjacent red and green (IdU) tracts); (iii) new origin firing (IdU/green tracts only). In the absence of HU, there was no statistically significant difference between any of these replication parameters in cells expressing WT RAD51 or K58/64R RAD51 protein ( Fig. 3b ). In contrast, following a 24-h exposure to HU, there was a significant change in the proportion of forks that remained stalled or were able to restart. For the K58/64R RAD51-expressing cells, a smaller proportion of replication forks were irreversibly stalled and a correspondingly greater proportion of forks successfully re-initiated DNA synthesis compared with cells expressing WT RAD51 ( Fig. 3b ). Although new origin firing also appeared suppressed in the K58/64R RAD51 cells compared with the control cells, this difference did not reach statistical significance. Equivalent results were also observed in K58/64 RAD51-expressing cells in which the endogenous RAD51 was depleted using an siRNA targeting the 3′-UTR of RAD51 ( Supplementary Fig. 3 ). 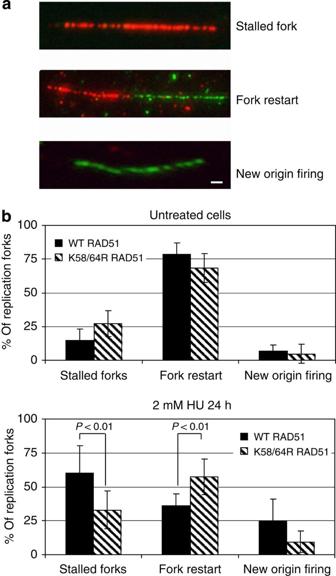Figure 3: Ubiquitylation on RAD51 influences replication fork restart. (a) Representative pictures of a stalled fork, fork restart and new origin firing from cells exposed to 2 mM HU for 24 h. DNA synthesis occurring before or after HU treatment was stained as red and green tracts, respectively. Scale bar, 1 μm (white). (b) Quantification of the percentage of replicons with stalled forks, re-started forks or newly fired origins for cells expressing WT RAD51 (black bars) or K58/64R RAD51 (hatched bars). The upper panel shows untreated cells and the lower panel shows cells exposed to HU for 24 h. The means are shown for two independent experiments. Where significant (P<0.01),P-values are indicated. At least 180 forks for each cell line were quantified and the differences in the distributions of stalled forks and fork restart after HU treatment were evaluated statistically using an unpairedt-test. Error bars represent s.d. Figure 3: Ubiquitylation on RAD51 influences replication fork restart. ( a ) Representative pictures of a stalled fork, fork restart and new origin firing from cells exposed to 2 mM HU for 24 h. DNA synthesis occurring before or after HU treatment was stained as red and green tracts, respectively. Scale bar, 1 μm (white). ( b ) Quantification of the percentage of replicons with stalled forks, re-started forks or newly fired origins for cells expressing WT RAD51 (black bars) or K58/64R RAD51 (hatched bars). The upper panel shows untreated cells and the lower panel shows cells exposed to HU for 24 h. The means are shown for two independent experiments. Where significant ( P <0.01), P -values are indicated. At least 180 forks for each cell line were quantified and the differences in the distributions of stalled forks and fork restart after HU treatment were evaluated statistically using an unpaired t -test. Error bars represent s.d. Full size image RAD51 ubiquitylation controls subcellular localization It has been reported that both mouse ES cells lacking FBH1 helicase function and FBH1-depleted human cells show increased levels of RAD51 nuclear foci [15] . We analysed, therefore, whether ubiquitylation of RAD51 was important for regulating the subcellular localization of RAD51. For this, we treated cells with 2 mM HU for 24 h, as we had seen the most dramatic differences in the levels of DSBs using this regimen. Using fluorescence microscopy, we found a reduced level of the ubiquitylation-resistant RAD51 localized to the cytoplasm, as compared with cells expressing the WT RAD51 protein ( Fig. 4a,b ; P <0.05 using an unpaired t -test). Consistent with this, a correspondingly increased number of RAD51 nuclear foci were evident in the K58/K64 RAD51-expressing cells ( Fig. 4c ; P <0.05 using an unpaired t -test, compared with the WT RAD51 cells). Importantly, these experiments were performed without permeabilizing the cell membrane before fixing the cells, to preserve the cytoplasmic RAD51 signal. Following depletion of the endogenous RAD51 messenger RNA, the cells were also analysed for the subcellular localization of the transfected RAD51. As shown in Supplementary Fig. 4a , there was a substantial difference in the percentage of cells expressing RAD51 in the cytoplasm, with an approximately tenfold greater proportion of cytoplasmic RAD51 seen in the cells expressing WT RAD51 compared with those expressing K58/64R RAD51, confirming the data presented in Fig. 4a–c . Consistent with these immunofluorescence data, we demonstrated that the K58/64R RAD51 was approximately equally distributed between the chromatin and soluble fractions, whereas the WT RAD51 was strongly concentrated in the soluble fraction ( Fig. 4d ). This localization bias was not affected by depleting the endogenous RAD51 with an siRNA targeting the 3′-UTR of RAD51 ( Supplementary Fig. 4b ). 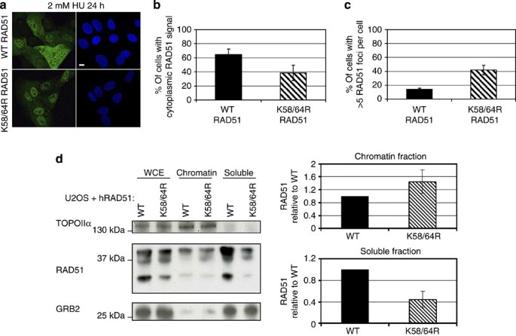Figure 4: Ubiquitylation of RAD51 regulates its intracellular localization. (a) Examples of RAD51 staining (green) in WT RAD51- and K58/64R RAD51-expressing cells after treatment with 2 mM HU for 24 h. Nuclei were stained with DAPI (blue). Scale bars, 10 μm (white). (b) The means of the percentage of cells showing cytoplasmic RAD51 staining are shown for three independent experiments. At least 50 cells for each cell line were quantified in each experiment. (c) The means of cells showing more than five RAD51 nuclear foci are shown for three independent experiments. At least 50 cells for each cell line were quantified in each experiment. (d) WT and K58/64R RAD51-expressing cells were exposed to 2 mM HU for 24 h. Whole-cell extracts (WCE), chromatin-bound proteins and soluble proteins were separated by SDS–PAGE and the samples were western blotted with an anti-TOPIIαantibody (a marker for chromatin bound proteins), an anti-RAD51 antibody, or an anti-GRB2 antibody (a marker for cytoplasmic proteins). In the right hand panels, the relative amount of RAD51 WT (black bars; set at 1 in each case) and K58/64R RAD51 (hatched bars) in the chromatin (upper) and soluble (lower) fractions were quantified by using ImageJ software. The means are shown for three independent experiments. Error bars represent s.d. Figure 4: Ubiquitylation of RAD51 regulates its intracellular localization. ( a ) Examples of RAD51 staining (green) in WT RAD51- and K58/64R RAD51-expressing cells after treatment with 2 mM HU for 24 h. Nuclei were stained with DAPI (blue). Scale bars, 10 μm (white). ( b ) The means of the percentage of cells showing cytoplasmic RAD51 staining are shown for three independent experiments. At least 50 cells for each cell line were quantified in each experiment. ( c ) The means of cells showing more than five RAD51 nuclear foci are shown for three independent experiments. At least 50 cells for each cell line were quantified in each experiment. ( d ) WT and K58/64R RAD51-expressing cells were exposed to 2 mM HU for 24 h. Whole-cell extracts (WCE), chromatin-bound proteins and soluble proteins were separated by SDS–PAGE and the samples were western blotted with an anti-TOPII α antibody (a marker for chromatin bound proteins), an anti-RAD51 antibody, or an anti-GRB2 antibody (a marker for cytoplasmic proteins). In the right hand panels, the relative amount of RAD51 WT (black bars; set at 1 in each case) and K58/64R RAD51 (hatched bars) in the chromatin (upper) and soluble (lower) fractions were quantified by using ImageJ software. The means are shown for three independent experiments. Error bars represent s.d. Full size image RAD51 ubiquitylation does not prevent BRCA2 interaction The BRCA2 protein has been shown to interact with and stimulate RAD51 loading onto RPA-coated ssDNA [29] , [30] , [31] , [32] . Therefore, we tested the proposal that RAD51 ubiquitylation might interfere with its ability to interact with BRCA2. To do this, we analysed the co-immunoprecipitation of RAD51 or K58/64 RAD51 with BRCA2 in cells in which the endogenous RAD51 had been depleted. As shown in Fig. 5 , the WT and K58/64R RAD51 proteins were equally effective at co-immunoprecipitating endogenous BRCA2, suggesting that ubiquitylation of RAD51 does not affect the RAD51–BRCA2 interaction. 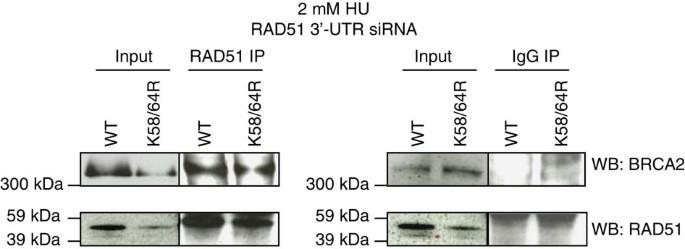Figure 5: RAD51 ubiquitylation does not disrupt the RAD51–BRCA2 interaction. WT RAD51- and K58/64R RAD51-expressing cells were treated with an siRNA targeting the 3’-UTR of RAD51 for 72 h, followed by a treatment with 2 mM HU for 24 h. Whole-cell extracts of WT RAD51- and K58/64R RAD51-expressing U2OS cells were incubated with anti-RAD51 (left panel) or anti-IgG control (right panel) antibodies. Precipitated proteins were separated by SDS–PAGE and the samples were western blotted with anti-BRCA2 and anti-RAD51 antibodies, as indicated. Figure 5: RAD51 ubiquitylation does not disrupt the RAD51–BRCA2 interaction. WT RAD51- and K58/64R RAD51-expressing cells were treated with an siRNA targeting the 3’-UTR of RAD51 for 72 h, followed by a treatment with 2 mM HU for 24 h. Whole-cell extracts of WT RAD51- and K58/64R RAD51-expressing U2OS cells were incubated with anti-RAD51 (left panel) or anti-IgG control (right panel) antibodies. Precipitated proteins were separated by SDS–PAGE and the samples were western blotted with anti-BRCA2 and anti-RAD51 antibodies, as indicated. Full size image The UvrD family of DNA helicases appears to play a number of roles in the cellular response to both DNA damage and DNA replication stress. Some, but not all, eukaryotes express a specialized UvrD family member, FBH1, which combines a helicase function with the ability to ubiquitylate target proteins. Previous results from analysis of S. pombe , mouse and human cells have indicated that the helicase activity of FBH1 is an important regulator of the function of RAD51. The data presented here indicate that RAD51 is also a substrate for the F-box-mediated E3 ubiquitin ligase action of FBH1. Analysis of the FBH1-mediated ubiquitylation reaction suggests that RAD51 can be targeted on several lysine residues in vitro , although each protein is rarely modified more than once. The apparent monoubiquitylation of RAD51 generated by FBH1 is different from the polyubiquitylation events more usually seen with other SCF complexes. Among the five lysine residues being ubiquitylated in vitro by FBH1, some lie within domains of the protein that are critical for function. K58 is adjacent to E59, which is involved in the interaction with the BRC4 peptide of BRCA2 (ref. 33 ). Although we showed that the WT and K58/64R RAD51 proteins were equally effective at co-immunoprecipitating endogenous BRCA2, there is still a possibility that ubiquitylation of K58 might affect the RAD51–BRCA2 interaction under some circumstances. K64 has also been shown to be crucial in binding to both ssDNA and double-stranded DNA [34] . Similarly, K285 is a part of the ssDNA-binding loop 2 domain [35] . Ubiquitylation on K64 and K285 might, therefore, affect the RAD51–DNA interaction. In contrast, K156 lies within the ATPase core domain [35] . Ubiquitylation on K156 could possibly affect ATP binding and hydrolysis. The consequences of ubiquitylation on K107 remain unknown, as this residue does not seem to lie within any functional domain. We focused on analysis of two adjacent lysine residues in the non-catalytic N-terminal domain of RAD51, because the mass spectrometry data indicated that these were quantitatively by far the most important. Consistent with this, we found that the double K58/64R mutant was only very poorly ubiquitylated in vitro by the SCF FBH1 complex. To define whether ubiquitylation of K58 and K64 of RAD51 plays a role in the regulation of RAD51’s function in DNA repair or DNA replication, we compared the response of cells expressing either ectopic WT RAD51 or K58/64R RAD51 with a prolonged exposure to HU. We found several differences between these two transfected cell populations; most notably, the nuclear accumulation of K58/64R RAD51 was more prominent than it was with WT RAD51 following exposure to HU, and this was accompanied by enhanced HU resistance, a reduced level of HU-induced DSBs and hyperrecombination. These data support the model whereby ubiquitylation of RAD51 by FBH1 does not function to trigger RAD51 turnover by proteolysis, as is seen with several SCF-mediated ubiquitylation events, but rather serves to regulate the subcellular localization of RAD51. This suggests a potentially new paradigm for how SCF proteins can regulate target protein function. Nevertheless, our analyses would not detect the proteolytic removal of a small fraction of cellular RAD51 that exists, for example, at a very specific nuclear location. A previous study did observe that RAD51 is degraded via ubiquitylation, in a reaction that is regulated by RAD51C [36] . However, we found equivalent RAD51 protein levels in WT and K58/64R RAD51-expressing cells. On the other hand, it has also been reported that FBH1 is recruited to DNA replication and DNA damage sites by proliferating cell nuclear antigen (PCNA) [37] . Interestingly, FBH1 can itself be ubiquitylated (by CRL4 Cdt2 ), which leads to FBH1 degradation [37] . Moreover, ubiquitylation of FBH1 modulates its interaction with RAD51 (ref. 38 ). Therefore, the relationship between FBH1 and RAD51 is probably controlled by multiple ubiquitylation events. There are a number of striking parallels between the phenotype of mammalian cells expressing the ubiquitylation-resistant form of RAD51 and those carrying a deletion in the helicase domain of FBH1. Our previous analysis of a mouse ES cell line with an internal deletion in the Fbh1 helicase domain showed that these cells are HU resistant, hyperrecombinogenic and less prone to accumulate DSBs following replication stress [23] , all phenotypes reported here for the K58/64R RAD51-expressing cells. In the mouse mutant cells, RAD51 nuclear staining was prominent, even without exogenous DNA damage/replication blockade. In the current work, the differences apparent following manipulation of the ubiquitylation status of RAD51 were only seen following replication stress. Nevertheless, the most straightforward explanation for these data is that the helicase and F-box functions of FBH1 operate together to regulate the same protein target or targets (see model in Fig. 6 ). Our data indicate that one key target in human cells is RAD51, but do not exclude the possibility that other targets for FBH1 exist. However, the fact that we can dominantly change the cellular response to HU simply by expressing a form of the proposed target protein that has altered ubiquitylation argues strongly that RAD51 is an important target for FBH1 during the cellular response to dNTP depletion and replication blockade. As ssDNA is commonly found adjacent to perturbed DNA replication sites, we tested the effect of ssDNA on the ubiquitylation reaction. Although we found that the presence of ssDNA does not alter the efficiency of the FBH1-mediated ubiquitylation reaction, it nevertheless might affect the specificity of the reaction in vivo . 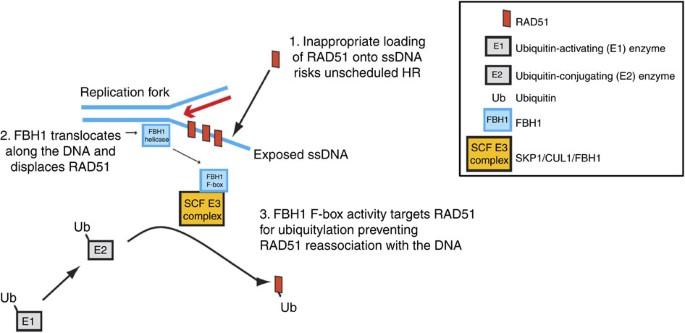Figure 6: Model for the proposed action of FBH1 at stalled DNA replication forks. Relevant proteins are shown, as indicated in the key. We propose that FBH1 translocates along DNA, where a physical interaction with RAD51 causes the dissociation of RAD51 from the developing nucleofilaments. Following this displacement of RAD51, the SCFFBH1targets RAD51 for ubiquitylation, preventing its re-association with the DNA. Figure 6: Model for the proposed action of FBH1 at stalled DNA replication forks. Relevant proteins are shown, as indicated in the key. We propose that FBH1 translocates along DNA, where a physical interaction with RAD51 causes the dissociation of RAD51 from the developing nucleofilaments. Following this displacement of RAD51, the SCF FBH1 targets RAD51 for ubiquitylation, preventing its re-association with the DNA. Full size image Protein purification E. coli expressing recombinant human RAD51 protein were lysed and sonicated in lysis buffer (0.1 M Tris-HCl pH 8, 2 mM EDTA, 5% glycerol, 0.5 mM dithiothreitol (DTT), 0.2 mg ml −1 phenylmethylsulfonyl fluoride and 0.1% Triton X-100). The soluble protein fraction was dialysed against spermidine buffer (20 mM Tris-acetate pH 7.5, 7 mM spermidine-NaOH and 0.1 mM DTT). Precipitates were collected and dissolved in P100 buffer (0.1 M potassium phosphate pH 6.8, 0.1 M KCl, 10% glycerol and 0.5 mM DTT) and were then loaded onto a hydroxyapatite column (Bio-Rad). Bound proteins were eluted with H buffer (0.1 M KCl, 10% glycerol and 0.5 mM DTT, containing a gradient of 0.1–0.8 M potassium phosphate pH 6.8). Fractions containing RAD51 were pooled and dialysed against R buffer (20 mM Tris-HCI pH 8, 1 mM EDTA, 0.5 mM DTT, 10% glycerol) containing 0.1 M KCl. Lysate was then loaded onto a heparin sepharose column (GE Healthcare) and eluted in R buffer with a linear gradient of 0.1–0.8 M KCl. Fractions containing RAD51 were again pooled and dialysed against R buffer containing 0.1 M KCl. Eluate was then loaded onto a mono-Q column (GE Healthcare) and eluted in R buffer with a linear gradient of 0.1–0.8 M KCl. Eluate was concentrated, dialysed against storage buffer (20 mM Tris-acetate pH 8, 0.2 M potassium acetate, 10% glycerol, 1 mM EDTA and 0.5 mM DTT) and stored at −80 °C [7] . S. cerevisiae expressing histidine-tagged human BLM protein were lysed in buffer A (50 mM HEPES-OH pH 7.2, 250 mM KCl, 10% glycerol and EDTA-free protease inhibitor (Roche)). The soluble protein fraction was subjected to nickel chelate affinity chromatography. The bound protein was eluted in buffer A containing 250 mM EDTA with an imidazole gradient of 50–1,500 mM. Fractions containing BLM were dialysed against buffer A containing 1 mM EDTA, 1 mM 2-mercaptoethanol and 0.1 mM phenylmethylsulfonyl fluoride, and stored at −80 °C [39] . Purified FANCD2 was a kind gift from Dr J.-Y. Masson. Purified RPA was a kind gift from Dr Pavel Janscak. To purify the SCF FBH1 complex, the FBH1 cDNA was obtained from an IMAGE clone library and was sub-cloned into pFastBac HT-A (Life Technologies, Inc.). The plasmid was then transformed into E. coli DH10Bac and recombinant bacmids were isolated for baculovirus preparation. Recombinant bacmids were transfected into SF21 cells to produce virus stocks. Baculoviruses encoding glutsthopne S -transferase (GST)-tagged SKP1, CUL1 and ROC1 were kindly provided by Dr Pavel Janscak. For SCF FBH1 complex production, SF21 cells were infected with the mixture of four recombinant baculoviruses: His-tagged FBH1, GST-tagged SKP1, and untagged CUL1 and ROC1, and the cells were incubated for 3 days. The infected SF21 cells were harvested and washed twice with ice-cold PBS. Cells were then lysed using lysis buffer (50 mM sodium phosphate buffer (pH7.4), 300 mM NaCl, 1 mM EDTA, 2 mM β-mercaptoethanol, 10% glycerol, 0.1% Nonidet P-40, Proteinase inhibitor complete (Roche)) for 1 h on ice. The lysate was clarified by centrifugation (Beckman, 70Ti, 70,000 g , 4 °C, 1 h) and the supernatant was subsequently incubated with glutathione sepharose resin (GE healthcare) for 3 h. After the incubation, the resin was transferred to a disposable column (BioRad) and was washed with 20 bed volumes of GST-wash buffer (50 mM sodium phosphate buffer (pH7.4), 300 mM NaCl, 10% glycerol, 2 mM β-mercaptoethanol). Bound proteins were eluted using GST-elution buffer (50 mM sodium phosphate buffer (pH 7.4), 20 mM glutathione, 300 mM NaCl, 10% glycerol, 2 mM β-mercaptoethanol). The eluted fractions were incubated with Ni-NTA agarose (QIAGEN) overnight. The resin was transferred to a disposable column and was washed sequentially with HS wash buffer (50 mM sodium phosphate buffer (pH7.4), 500 mM NaCl, 10% glycerol, 1 mM β-mercaptoethanol, 10 mM imidazole) and IM wash buffer (50 mM sodium phosphate buffer (pH7.4), 300 mM NaCl, 10% glycerol, 1 mM β-mercaptoethanol, 25 mM imidazole). Bound proteins were eluted with HIS-elution buffer (50 mM sodium phosphate buffer (pH7.4), 300 mM NaCl, 10% glycerol, 1 mM β-mercaptoethanol, 300 mM imidazole). Aliquots were frozen in liquid N 2 and stored at −80 °C. In vitro ubiquitylation assays A complete ubiquitylation reaction (10 μl), containing ubiquitylation buffer (50 mM HEPES-NaOH pH 7.5, 100 mM NaCl, 10 mM MgCl 2 , 5 mM ATP, 0.1 mM DTT), 100 nM ubiquitin activating enzyme (Boston Biochem), 500 nM UbcH5a (Boston Biochem), 8 μM untagged or HA-tagged ubiquitin (Boston Biochem), 20 nM purified RAD51 and 5 ng μl −1 SCF FBH1 , was incubated at 37 °C for the indicated times. The reactions were terminated by incubation with 10 μl stop buffer (100 mM Tris-HCl pH 8, 5 mM EDTA pH 8.0, 0.2% SDS, 200 mM NaCl, 200 μg ml −1 proteinase K) at 65 °C for 15 min. The reaction products were analysed by SDS–PAGE followed by western blotting with antibodies against RAD51 (1:200, Abcam ab1837), BLM (1:1,000, Abcam ab476), FANCD2 (1:200, Santa Cruz sc28194), RPA14 (1:1,000, Tebu-bio GTX70238), RPA34 (1:1,000, Abcam ab2175) or RPA70 (1:1,000, NeoMarkers MS-692-P) using standard methods. Where indicated, 25 μg ml −1 ssDNA was included in the reaction. To test the ability of different E2 enzymes to support the ubiquitylation reaction, 500 nM Cdc34 or UbcH6 was used instead of UbcH5a. Cdc34 was also tested at the same concentration in combination with UbcH5, to assess whether this enhanced the reaction efficiency, as has been suggested previously [40] . Nedd8 (25 μM)- and Nedd8-activating enzyme (100 nM) were tested based on reports that SCF-mediated polyubiquitylation is activated by conjugation of Nedd8 to human CUL1 (refs 41 , 42 ), probably via conformational changes in CUL1 (ref. 43 ). Immunoprecipitation of FBH1 and RAD51 Two hundred nanograms of GST (Santa Cruz) or GST-FBH1 was incubated with 4 pmol WT or K58/64R RAD51 in 500 μl binding buffer (10 mM Tris-HCl pH8, 150 mM NaCl, 1 mM EDTA and 0.2% TrintonX-100) at 4 °C for 15 min. Forty microlitres of Glutathione Sepharose (GE Healthcare) was added and the protein mixture was incubated at 4 °C for 1 h. The sepharose was collected and washed with the binding buffer five times. The sepharose was then boiled with the sample buffer (0.4% SDS, 2% glycerol, 12 mM Tris-HCl pH 6.8, 0.1% (w/v) bromophenol blue, 5% (w/v) β-mercaptoethanol) and the released proteins were analysed by using western blotting. Membranes were probed with antibodies against GST (1:200, Santa Cruz sc138) or RAD51 (1:1,000, Santa Cruz sc8349). Mass spectrometry-based analysis of RAD51 ubiquitylation Proteins were resolved by SDS–PAGE, followed by in-gel digestion with trypsin. Peptide fractions were analysed on a Orbitrap mass spectrometer (Velos, Thermo Scientific) equipped with a nanoflow HPLC system (Thermo Scientific) using a data-dependent method, dynamically choosing the ten most abundant precursor ions from the survey scan for higher energy collisional dissociation fragmentation. Survey scans were acquired at a resolution of 30,000 at m/z 400, while the resolution for higher energy collisional dissociation spectra was set to 7,500 at m/z 400 (ref. 44 ). Raw data files were analysed using MaxQuant software (version 1.2.2.9) [45] . Cell culture Human U2OS cells (obtained from the ATCC) were maintained in DMEM medium supplemented with 10% FCS and 2.4 mM glutamine. Cells were grown at 37 °C in a humidified atmosphere containing 5% CO 2 . Cells were transfected with plasmids expressing WT or mutated RAD51 under the control of cytomegalovirus promoter in vector pcDNA3 (a gift from Dr Fiona Benson) using standard techniques. Where indicated, cells were transfected with control siRNA (5′-UCUGUCGUUAGUGUCACCGGUCAUA-3′) or siRNA targeting the 3′-UTR of the RAD51 gene (5′-UCUUCCUGUUGUG ACUGCCAGGAUA-3′) for 72 h before HU treatment. To target the coding region of RAD51, the following siRNA was used: 5′-GCGACUCGCUGAUGAGUUUTT-3′. As a control, an siRNA with the following sequence was used: 5′-GCGGCUGUCG UAGAACUUUTT-3′. Pulsed-field gel electrophoresis Cells were treated with 2 mM HU for various times. After treatment, 10 6 cells were embedded into 0.9% agarose gel plugs using a CHEF disposable plug mould (BioRad). The plugs were incubated in lysis buffer (100 mM EDTA, 1% sodium lauryl sarcosine, 0.2% sodium deoxycholate, 1 mg ml −1 proteinase K) for 2 days and run in an 0.9% agarose gel using a Rotaphor apparatus (Biometra) [46] . The gel was then stained with ethidium bromide and the DNA was analysed using a Typhoon 9200 scanner (Amersham). Band intensities were quantified using ImageQuant 5.2 software. All experiments were performed at least three times. Clonogenic survival assays Cells were incubated in HU or Aphidicolin-containing medium for 24 h. After treatment, cells were washed with PBS and then grown in fresh medium for 8–10 days. Colonies were fixed, stained and counted using Coomassie solution (0.1% Coomassie Blue, 7% acetic acid, 50% methanol). All experiments were performed at least three times. DR-GFP recombination assay The recombination level in U2OS cells was measured by transfecting cells using electroporation (Gene Pulser Xcell, Bio-Rad) with the DSB recombination reporter (which generates an intact GFP gene following recombination) and an I- Sce I endonuclease expression vector. A red fluorescent protein expression vector was used as a control, to define transfection efficiency. Cells were analysed by flow cytometry for green/red fluorescence 3 days after transfection [28] . Immunofluorescence analysis Cells in DMEM medium were seeded onto glass coverslips at ~25% confluency. Twenty-four hours later, the cells were treated with 2 mM HU and were then incubated at 37 °C for 24 h. Cells were then fixed in 4% para -formaldehyde in PBS for 10 min, washed in PBS and were stored at 4 °C. After permeabilization with 0.1% TritonX-100 in PBS, the cells were washed in freshly made blocking buffer (0.15% glycine (w/v), 0.5% BSA (w/v) in PBS). Staining with primary antibody against RAD51 (1:200, Santa Cruz sc8349) was followed by further washes with 0.1% TritonX-100 in PBS and then incubation with secondary antibody conjugated with AF488 (1:800, Invitrogen A21206). The nuclei were counterstained with DAPI (Vector Laboratories) before the coverslips were sealed to glass slides. RAD51 staining patterns were visualized with a confocal laser scanning microscope (Zeiss LSM 710) and images were stored and analysed using Zeiss LSM Image Browser software. Separation of soluble and chromatin-associated proteins Cells were treated with 2 mM HU and incubated at 37 °C for 24 h. A pellet of ~2 × 10 6 cells was washed three times in PBS and then re-suspended in 250 μl freshly made protein buffer A (10 mM HEPES, 10 mM KCl, 1.5 mM MgCl 2 , 0.34 M sucrose, 10% glycerol, 1 mM DTT, 0.1% TritonX-100, protease inhibitor complete (Roche)) for 1 h at 4 °C. The sample was centrifuged at 200 g for 4 min at 4 °C and the supernatant was stored as the cytoplasmic soluble fraction. The pellet was washed three times in 200 μl Protein Buffer A, centrifuged at 180 g for 4 min at 4 °C before addition of 175 μl of freshly made protein buffer B (3 mM EDTA, 0.2 mM EGTA, 1 mM DTT, protease inhibitor complete (Roche)). Incubation continued for 1 h at 4 °C, followed by centrifugation at 300 g for 4 min at 4 °C. The supernatant was stored as the nuclear soluble fraction. The pellet was washed three times in 175 μl Protein Buffer B, centrifuged at 16,000 g for 1 min at 4 °C before the supernatant was discarded, and the pellet (chromatin-associated fraction) was resuspended and boiled in 175 μl Laemmli buffer (0.4% SDS, 2% glycerol, 12 mM Tris-HCl pH 6.8). For western blotting analysis, 10 × BFB-2-ME (0.1% (w/v) bromophenol blue, 5% (w/v) β-mercaptoethanol) was added, the samples were boiled, and the cytoplasmic and nuclear soluble fractions were combined. Membranes were probed with antibodies against RAD51 (1:1,000, Abcam ab1837), TOPOIIα (1:1,000, Santa Cruz sc5347) or GRB2 (1:1,000, BD Transduction lab 610112). Uncropped gel scans can be found in Supplementary Fig. 5 . DNA fibre analysis U2OS cells were pulse-labelled with 50 μM CldU for 20 min. The cells were rinsed with fresh medium and were incubated with 2 mM HU for 24 h. Cells were rinsed with medium again and pulse labelled with 500 μM IdU for 1 h. For untreated cells, the HU incubation was omitted. Labelled cells were harvested and DNA fibres were spread on glass slides [47] . DNA fibres were denatured with 2.5 M hydrochloric acid for 90 min and then rinsed with freshly made blocking buffer (0.15% glycine (w/v), 0.5% BSA (w/v) in PBS). CldU and IdU were detected by incubating slides with primary antibodies (1:40, Abcam ab6326 and 1:2, Becton Dickinson 347580, respectively). DNA fibres were washed with blocking buffer again, and then incubated with secondary antibodies conjugated with AF568 (1:200, Invitrogen A11077) or AF488 (1:200, Invitrogen A21200). At least 180 replication structures for each analysis were scored using a Nikon Eclipse 80i microscope equipped with ACT-1 software. Immunoprecipitation of RAD51 and BRCA2 Cells were treated with 2 mM HU and incubated at 37 °C for 24 h. Cells were washed three times in cold PBS and then scraped in 1 ml RIPA buffer (50 mM Tris pH 7.5, 150 mM NaCl, 1% TrintonX-100, 0.1% sodium deoxycholate, 1 mM EDTA, 5 mM β-glycerophosphate, 1 mM sodium orthovanadate and 5 mM sodium fluoride, protease inhibitor complete (Roche)). Cells were lysed in RIPA buffer at 4 °C for 30 min. The lysate was sonicated briefly and then incubated with RAD51 antibody (1:40, Santa Cruz sc8349) or rabbit IgG antibody (1:80, Santa Cruz sc2027) at 4 °C for 1 h. Twenty-five microlitres of protein G Sepharose (Invitrogen) was added to the lysate and incubated at 4 °C for 1 h. The sepharose was collected and washed with the RIPA buffer three times. The sepharose was then boiled with the sample buffer (0.4% SDS, 2% glycerol, 12 mM Tris-HCl pH 6.8, 0.1% (w/v) bromophenol blue, 5% (w/v) β-mercaptoethanol) and analysed by using western blotting. Membranes were probed with antibodies against BRCA2 (1:1,000, Abcam ab123491) or RAD51 (1:1,000, Santa Cruz sc8349). How to cite this article : Chu, W. K. et al. FBH1 influences DNA replication fork stability and homologous recombination through ubiquitylation of RAD51. Nat. Commun. 6:5931 doi: 10.1038/ncomms6931 (2015).